Oxygen-driven anisotropic transport in ultra-thin manganite films Transition metal oxides have a range of unique properties due to coupling of charge, spin, orbital and lattice degrees of freedom and nearly degenerate multiple ground states. These properties make them interesting for applications and for fundamental investigations. Here we report a new phase with abnormal transport anisotropy in La 0.7 Sr 0.3 MnO 3 ultra-thin films under large tensile strain. This anisotropy is absent in films under smaller tensile strain or compressive strain. Furthermore, thickness and magnetic-field-dependent experiments suggest that the tensile-strain-induced two-dimensional character is crucial for the observed phenomena. X-ray absorption spectroscopy results indicate that this anisotropy is likely driven by O 2 p orbital, which hybridizes with Mn 3 d . Ab initio calculations confirm this result. Our results may help to understand the anisotropic transport behaviour observed in other systems. The emergence of exotic electronic phases from intricate coupling of charge, spin, orbital and lattice degrees of freedom has been a central theme of research in modern condensed matter physics [1] , [2] , [3] . Among all the systems studied, complex oxides that contain 3 d orbital transition metals are of particular importance for both fundamental study and applications. It is well known that the physical properties of transition metal oxides depend strongly on the occupancy of Mn 3 d orbitals [4] , [5] , [6] , [7] , [8] , [9] , [10] , [11] . However, the effect of O 2 p orbital has attracted much less attention so far. Bulk La 0.7 Sr 0.3 MnO 3 (LSMO) is a large-bandwidth material with ferromagnetic (FM) metallic ground state and its physical properties can be described successfully by the double-exchange mechanism [12] . By depositing LSMO films on different substrates, epitaxial strain ranging from compressive to tensile can be induced ( Fig. 1a ). Here, we report pronounced in-plane transport anisotropy in highly strained ultra-thin LSMO films at low temperature. X-ray absorption spectroscopy (XAS) results indicate that this anisotropy is likely driven by O 2 p orbital and its hybridization with Mn 3 d , in connection with the strong correlations in the highly tensile-strained LSMO film. This is yet another example of exotic electronic phase induced by strong charge–spin–orbital–lattice coupling in transition metal oxides. 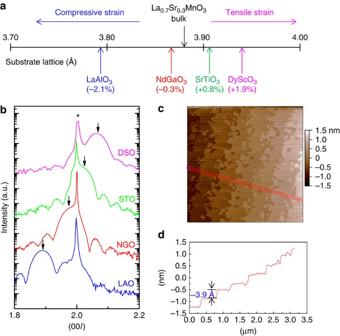Figure 1: Properties of LSMO on different substrates. (a) Lattice mismatch between LSMO and the substrates used in this study: −2.1% for LAO, −0.3% for NGO, +0.8% for STO and +1.9% for DSO. (b) XRD L scans around the (002)pcpeaks for 8 nm LSMO films on various substrates. The stars (*) and arrows (↓;) indicate the substrates and LSMO (002)pcpeaks, respectively. Clear Kiessig fringes indicate the high quality of the films. (c) Topography image of the 8 nm LSMO film on DSO substrate. Scan range is 3 μm × 3 μm. (d) Cross-sectional profile, averaged over the red rectangular box inFig. 1c, showing 1 unit cell (~3.9 Å) high steps. Figure 1: Properties of LSMO on different substrates. ( a ) Lattice mismatch between LSMO and the substrates used in this study: −2.1% for LAO, −0.3% for NGO, +0.8% for STO and +1.9% for DSO. ( b ) XRD L scans around the (002) pc peaks for 8 nm LSMO films on various substrates. The stars (*) and arrows (↓;) indicate the substrates and LSMO (002) pc peaks, respectively. Clear Kiessig fringes indicate the high quality of the films. ( c ) Topography image of the 8 nm LSMO film on DSO substrate. Scan range is 3 μm × 3 μm. ( d ) Cross-sectional profile, averaged over the red rectangular box in Fig. 1c , showing 1 unit cell (~3.9 Å) high steps. Full size image Thin film growth and transport measurements We have deposited high-quality epitaxial LSMO thin films using pulsed laser deposition on (001) pc -oriented LaAlO 3 (LAO), (110) o -oriented NdGaO 3 (NGO), (001) c -oriented SrTiO 3 (STO) and (110) o -oriented DyScO 3 (DSO) substrates (the subscripts ‘o’, ‘c’ and ‘pc’ represent orthorhombic, cubic and pseudocubic structures, respectively), all of which have pseudocubic lattice constants close to that of LSMO (see Methods for details). Figure 1b shows the XRD patterns of 8 nm LSMO films on these substrates. The arrows indicate the (002) pc peak of LSMO, which shifts from the left of substrate peak to the right, indicating that the strain changes from compressive to tensile. Figure 1c shows the topography image of the 8 nm LSMO film on DSO. The unit cell level steps clearly suggest step flow growth mode of the films ( Fig. 1d ). The films are fully strained to the substrate, which is confirmed by synchrotron reciprocal space mappings (see Supplementary Fig. S1 and Supplementary Note 1 for details). The results reveal that the 8 nm LSMO on DSO has c =3.826 Å and a tetragonal distortion of c / a =0.968. According to the calculated temperature–strain phase diagram [5] , fully strained LSMO film on LAO and DSO have C -type and A -type antiferromagnetic (AFM) ground states at low temperature, respectively, whereas those grown on NGO and STO have the FM ground state. Indeed, this is confirmed by the temperature dependence of in-plane resistivity as shown in Fig. 2a , which is consistent with previous reports [6] , [7] , [8] . Under relatively small compressive (on STO) or tensile (on NGO) strain, the LSMO thin film shows metallic behaviour with slightly reduced Curie temperature. Under large compressive or tensile strains (on LAO and DSO), it becomes insulating. 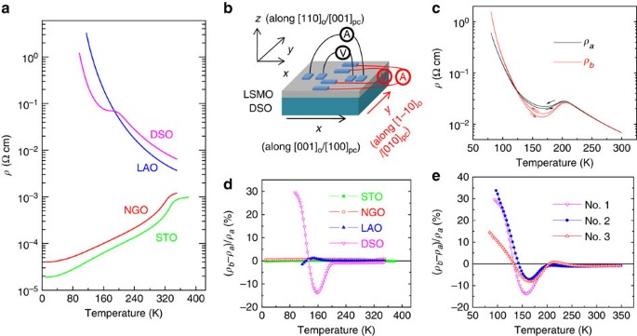Figure 2: In-plane resistivity anisotropy of LSMO on DSO substrate. (a) Temperature dependence of resistivity of 8 nm LSMO thin films on different substrates under zero magnetic field. (b) Schematic illustration of the experimental set-up used to measure the in-plane resistivity of the LSMO thin films along the two orthogonal directions (xandy). The samples are square with a side length of 5 mm. The Pt electrodes are 0.4 mm × 0.8 mm. (c) Resistivity versus temperature curves for 9.6 nm LSMO on DSO along the two channels during cooling and heating processes. A hysteresis is observed in the intermediate region indicating two-phase coexistence; while it is absent in the low- and high-temperature regions. (d) The in-plane resistivity anisotropy, (ρb–ρa)/ρa, of 8 nm LSMO thin films on different substrates. Note that only the film on DSO under large tensile strain shows pronounced resistivity anisotropy. (e) The anisotropy versus temperature curves of three 8 nm LSMO films on DSO, confirming the repeatability of the result. Note the switching of anisotropy sign from negative to positive upon cooling. Figure 2: In-plane resistivity anisotropy of LSMO on DSO substrate. ( a ) Temperature dependence of resistivity of 8 nm LSMO thin films on different substrates under zero magnetic field. ( b ) Schematic illustration of the experimental set-up used to measure the in-plane resistivity of the LSMO thin films along the two orthogonal directions ( x and y ). The samples are square with a side length of 5 mm. The Pt electrodes are 0.4 mm × 0.8 mm. ( c ) Resistivity versus temperature curves for 9.6 nm LSMO on DSO along the two channels during cooling and heating processes. A hysteresis is observed in the intermediate region indicating two-phase coexistence; while it is absent in the low- and high-temperature regions. ( d ) The in-plane resistivity anisotropy, ( ρ b – ρ a )/ ρ a , of 8 nm LSMO thin films on different substrates. Note that only the film on DSO under large tensile strain shows pronounced resistivity anisotropy. ( e ) The anisotropy versus temperature curves of three 8 nm LSMO films on DSO, confirming the repeatability of the result. Note the switching of anisotropy sign from negative to positive upon cooling. Full size image In-plane transport anisotropy Interesting results are observed when the in-plane resistivity is measured along both of the orthogonal directions. The measurement set-up is shown schematically in Fig. 2b (the x , y and z directions are defined along the pseudocubic a , b and c directions. See Supplementary Fig. S2 for details). For the film grown on DSO, abnormal in-plane transport anisotropy is observed ( Fig. 2c ) and the resistivity along the longer a direction is lower, which has not been reported before. The resistivity anisotropy ( ρ b – ρ a )/ ρ a is ~30% at 95 K for the 8 nm film and it does not show saturation within our measurement range. More interestingly, there is a switch of easy axis (low resistivity axis) at ~130 K. This phenomenon is reproducible as shown in Fig. 2e for three samples. On the contrary, films grown on STO, NGO and LAO show negligible in-plane resistivity anisotropy ( Fig. 2d ). For the film on DSO, the hysteresis in the resistivity–temperature curves between ~130 K and 210 K obtained during cooling and heating suggest coexistence of two phases ( Fig. 2c ). It is likely that the anisotropy within this temperature range is the result of anisotropic nucleation and growth of the low temperature phase following the percolation theory. Such behaviour has been observed in other manganite systems, for example, Nd 0.5 Sr 0.5 MnO 3 (ref. 13 ) and La 0.325 Pr 0.3 Ca 0.375 MnO 3 (ref. 14 ). However, the new phenomenon here is the anisotropic resistivity at temperatures below 130 K, which does not show hysteresis between heating and cooling and suggests new phase with intrinsic anisotropy. To understand this phase, we have to start with the crystal structures of the substrates. STO has a cubic structure, thus no anisotropy is expected for the LSMO film grown on it. LAO has a rhombohedral structure, and the two in-plane lattice are equivalent in the pseudocubic unit cell, thus no anisotropy is expected either. NGO, on the other hand, has an orthorhombic structure with lattice constants of 5.428 Å (along [100] o ), 5.498 Å (along [010] o ), and 7.709 Å (along [001] o ) [15] . The NGO (110) o surface has a nearly square mesh with pseudocubic lattices of a =3.855 Å along [001] o and b =3.863 Å along [1–10] o direction, which leads to ~0.2% strain anisotropy in the LSMO films along the two orthogonal in-plane directions. We do not observe any anisotropy in the transport, indicating that the small strain difference alone is not enough to induce detectable changes in the electron hopping along these two directions. Note that the pseudocubic lattice constant of NGO is close to that of LSMO, so the overall strain is small (~ −0.3%). DSO has an orthorhombic structure similar to that of NGO with lattice constants of 5.442 Å (along [001] o ), 5.719 Å (along [010] o ) and 7.904 Å (along [001] o ) (ref. 15 ). The (110) o surface has pseudocubic lattices of a =3.952 Å along [001] o /[100] pc and b =3.947 Å along [1–10] o /[010] pc directions ( Fig. 2b ), resulting in ~1.9% overall tensile strain on LSMO with ~0.13% in-plane anisotropy. Theoretical calculation has shown that the in-plane Mn–O–Mn bond angle does not change much for c/a <1 (under tensile strain) [16] , so electrons are expected to hop more easily between atoms along the shorter axis with larger orbit overlapping. However, the resistivity along the shorter b axis is larger than that along the longer a axis at low temperature in LSMO on DSO, which is counterintuitive. Furthermore, negligible anisotropy is observed in films on NGO with even larger strain anisotropy (~0.2%), suggesting that the large over-tensile strain (~1.9%) for films on DSO may be crucial for the low-temperature transport anisotropy. The c/a of the ultra-thin LSMO film obtained from synchrotron reciprocal space mapping is about 0.968, which is right around the calculated FM to A -type AFM phase transition point [5] . If this occurs in our samples and the A -type AFM phase is related to the observed transport anisotropy, then perturbing it with external stimulus may lead to suppression of the transport anisotropy. We have conducted two experiments to test this prediction. First, as the AFM phase is stabilized by the large tensile strain from the substrate, by increasing the film thickness, it should gradually change to the bulk FM phase. This process will suppress the low-temperature phase and enlarge the negative anisotropy region that originates from the anisotropic percolation. Indeed, this is observed experimentally as shown in Fig. 3a,b . Increasing film thickness leads to a decrease of the switching temperature from negative to positive anisotropy, as shown in the inset of Fig. 3b . More interestingly, a magnetic field in the out-of-plane direction leads to similar effect as shown in Fig. 3c,d . This clearly demonstrates the strong spin–orbital–lattice coupling in these ultra-thin LSMO films and supports a low-temperature phase with spin aligned in-plane. Applying a magnetic field in the out-of-plane direction causes the Mn spins to cant so that they are partially aligned out-of-plane. This canting allows for some inter-plane hopping and reduces the confinement of carriers to the ab planes, again leading to suppression of the low-temperature phase. The critical temperature between the percolation and low-temperature-phase-dominated regions also decreases as shown in the inset of Fig. 3d . These two experiments confirm that the low temperature transport anisotropy is closely related to the tensile-strain-induced A -type AFM phase. However, what triggers the anisotropic transport is still unclear. 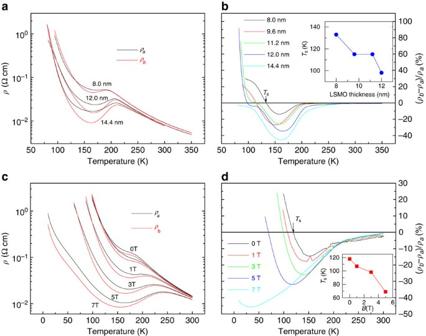Figure 3: Thickness and magnetic field dependences of resistivity and (ρb–ρa)/ρa. (aandb) The resistivity and (ρb–ρa)/ρaversus temperature curves for LSMO films on DSO with different thickness. Inset: thickness dependence of anisotropy switching temperature (Ts). (candd) The resistivity and (ρb–ρa)/ρaversus temperature curves under different magnetic fields for 9.6 nm LSMO films on DSO. Inset: magnetic field dependence ofTs. Figure 3: Thickness and magnetic field dependences of resistivity and ( ρ b – ρ a )/ ρ a . ( a and b ) The resistivity and ( ρ b – ρ a )/ ρ a versus temperature curves for LSMO films on DSO with different thickness. Inset: thickness dependence of anisotropy switching temperature ( T s ). ( c and d ) The resistivity and ( ρ b – ρ a )/ ρ a versus temperature curves under different magnetic fields for 9.6 nm LSMO films on DSO. Inset: magnetic field dependence of T s . Full size image To better understand the low-temperature phase of LSMO on DSO, we turn to its electronic structure. Recall that the c/a of the film on DSO is right around the calculated FM/ A -type AFM transition point. The large tensile strain may have profound effect on the Mn 3 d and O 2 p orbital occupancy, which can be revealed by element-specific XAS measurements. The XAS measurements using linearly polarized light are performed at the Mn L edges and O K edge (see Methods for details). The former is mainly dipole-allowed Mn 2 p →3 d transitions. Due to spin–orbit interaction of Mn 2 p , the core state splits the spectrum into two broad multiplets, the L 3 (Mn 2 p 3/2 →3 d ) edge at ~643 eV and the L 2 (Mn 2 p 1/2 →3 d ) edge at ~654 eV. From here, one can determine the 3 d occupancy of the Mn [9] , [17] . The later is dipole-allowed O 1 s →2 p transitions. Because the O 2 p hybridizes with transition metals, especially Mn 3 d , one can thus determine the importance of O 2 p as well as the hybridization of O 2 p with Mn 3 d and map the unoccupied states in a broad energy range [17] . The XAS results are shown in Fig. 4 . For Mn, the and orbitals have lobes pointing perpendicular and parallel to the pseudocubic ab plane ( xy plane), respectively. Their occupancy can be probed by linearly polarized light aligned to the out-of-plane ( E || c ) and in-plane ( E || a or b ) directions (inset of Fig. 4b ). 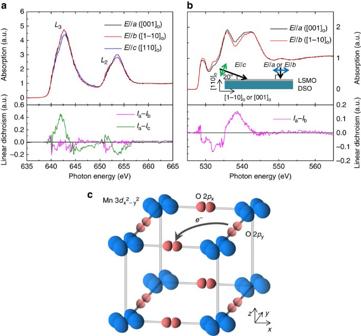Figure 4: XAS results and schematic orbitals diagram. (a) Mn L-edge XAS results and their linear dichroism at 80 K. (b) OK-edge XAS results and their linear dichroism at 80 K. (c) Schematic Mn 3dand O 2porbitals occupancy of LSMO on DSO near the Fermi level. The arrow indicates that some electrons transfer from O 2pxto 2pyorbital, enhancing the O 2p–Mn 3dhybridization and increasing the conductivity along the longeradirection in LSMO. For clarity, the less occupied Mnand O 2pzorbitals are not shown. Figure 4a shows the spectra obtained at the Mn L 3,2 -edges at 80 K. The spectra difference ( I a – I c ) implies a preferential occupancy of the orbital, which is in good agreement with the theoretically calculated result for LSMO film under tensile strain (see Supplementary Fig. S3 ) [9] . It is also consistent with orbital occupancy of Mn e g electrons in A -type AFM phase [4] , [5] . Unfortunately, because the DSO substrate has a very large paramagnetic signal, we could not conduct magnetometry measurement on our films [18] . However, Takamura et al . [6] has conducted X -ray magnetic circular dichroism measurements on similar samples and the results support A -type AFM phase. Figure 4: XAS results and schematic orbitals diagram. ( a ) Mn L-edge XAS results and their linear dichroism at 80 K. ( b ) O K -edge XAS results and their linear dichroism at 80 K. ( c ) Schematic Mn 3 d and O 2 p orbitals occupancy of LSMO on DSO near the Fermi level. The arrow indicates that some electrons transfer from O 2 p x to 2 p y orbital, enhancing the O 2 p –Mn 3 d hybridization and increasing the conductivity along the longer a direction in LSMO. For clarity, the less occupied Mn and O 2 p z orbitals are not shown. Full size image Next, we focus on the in-plane XAS results. The spectra difference ( I a – I b ) of Mn L-edge shows a very small anisotropy (~2% of the absorption peak intensity) between the a and b directions. Thus, the Mn 3 d orbital occupancy alone cannot account for the observed anisotropy in transport. On the other hand, the O K -edge spectra shows surprisingly strong anisotropy in the broad energy range from ~528 to ~543 eV, which is separated into two regions, one from ~528 to ~535 eV (the low-energy region) and the other from ~535 to ~543 eV (the high-energy region). First of all, it is known that hybridizations have important role at these energy regions [17] . In the low-energy region, the transitions are mainly to O 2 p –Mn 3 d hybridized states, whereas in the high-energy region the transitions are mainly to O 2 p –La 5 d /Sr 4 s hybridized states. Note that both regions are dominated by transitions to O 2 p . Secondly, we observe anomalous spectral weight transfer as large as 15% in such a broad energy range. As shown in previous studies, spectral weigh transfer is a fingerprint of strong correlations [19] , [20] , [21] , [22] . In this case, as seen in Fig. 4b , along the longer a direction there is a gain in spectra weight at the high-energy region of O 2 p –La 5 d /Sr 4 s -hybridized states, accompanied by a loss in spectral weight at the low-energy region of O 2 p –Mn 3 d -hybridized states. As XAS directly measures the unoccupied states, a loss (gain) in spectral weigh indicates a decrease (increase) in the unoccupied states of O 2 p , or in other words, along the a direction electrons in the O 2 p –La 5 d /Sr 4 s -hybridized states are transferred to the O 2 p –Mn 3 d -hybridized states, and thus the electrons in the O 2 p –Mn 3 d -hybridized states increase accordingly. Anomalous spectral weight transfer in such a broad energy range has been observed in other La 1– x Ca x MnO 3 (ref. 22 ) and attributed to oxygen [23] . Therefore, from polarized XAS results, we conclude that between the a and b directions: (1) there are more electrons occupying the O 2 p states along the a direction; (2) the O 2 p orbitals have important role for the observed transport anisotropy ( Fig. 4c ); and (3) hybridizations and strong correlations also contribute to the observed phenomenon. To better understand the XAS results and its connection to the transport, we conducted first principles calculations using Vienna Ab-initio Simulation Package (VASP) (see Methods for details). The supercell used in the calculations is shown in Fig. 5a . 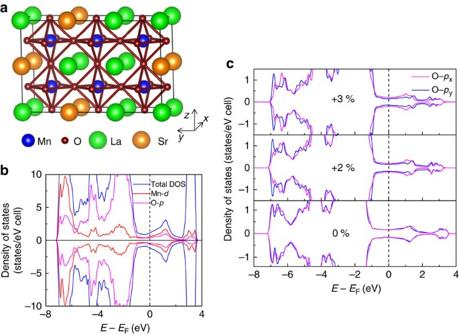Figure 5: Results of first-principles calculations. (a) The supercell used for calculations is La4Sr2Mn6O18(1 × 3 × 2) with experimental lattice constants:a=3.952 Å,b=3.947 Å andc=3.788 Å. (b) DOS obtained using GGA+U=6 eV. (c) DOS of O-px(pink lines) and O-py(blue lines) orbitals under various strain anisotropies with fixedydirection lattice constant (b=3.947 Å). Figure 5b shows the density of states of LSMO. It is found that both Mn 3 d and O 2 p orbitals contribute to the density of states significantly at the Fermi level ( Fig. 5b ). What is more interesting is that the occupancy of O 2 p x and 2 p y orbitals is affected by strain. As the tensile strain along x direction increases, the contribution to density of states at Fermi level from O 2 p x increases ( Fig. 5c ). Even though the strain anisotropy used in the calculations is significantly larger than that in the film, the trend is consistent with our XAS observation, supporting the significant role of O 2 p orbital in the transport anisotropy. However, note that the anisotropic occupancy of p x and p y orbitals alone does not lead to the anisotropic transport observed. In fact, our first principles calculations on over-all unstrained LSMO (but with an a , b lattice anisotropy of 3%) reveals similar trend in the p x and p y orbital occupancy (see Supplementary Fig. S4 and Supplementary Note 2 ). This again indicates that the large tensile-strain-induced A -type AFM phase is crucial to the observed transport anisotropy. Further study is needed to clarify the underlying physics. Figure 5: Results of first-principles calculations. ( a ) The supercell used for calculations is La 4 Sr 2 Mn 6 O 18 (1 × 3 × 2) with experimental lattice constants: a =3.952 Å, b =3.947 Å and c =3.788 Å. ( b ) DOS obtained using GGA+ U =6 eV. ( c ) DOS of O- p x (pink lines) and O- p y (blue lines) orbitals under various strain anisotropies with fixed y direction lattice constant ( b =3.947 Å). Full size image To summarize, the large tensile strain generated by DSO substrate leads to preferred occupancy of the Mn orbital at low temperature which is consistent with the theoretically predicted A -type AFM phase. Abnormal in-plane transport anisotropy is observed in this low-temperature phase, where the resistivity along the a direction is lower despite a > b . Both the XAS study and first principles calculations suggest that the anisotropy is triggered by the preferred occupancy of the O 2 p x orbitals. Why does this only occur in films under large tensile strain is an open question and further study is needed. Sample growth High-quality epitaxial LSMO thin films are grown by pulsed laser deposition on atomically smooth (001) pc -oriented LAO, (110) o -oriented NGO, (001) c -oriented STO and (110) o -oriented DSO single-crystal substrates. The laser pulse (248 nm) energy density was ~2 J cm −2 and the repetition rate was 3 Hz. The growth was carried out under 200 mTorr oxygen partial pressure at 800 °C and the growth rate was ~0.8 nm min −1 . Structure characterization The samples were investigated by high-resolution XRD using the X -ray demonstration and development beamline at SSLS (Singapore Synchrotron Light Source). The diffractometer is the Huber 4-circle system 90000-0216/0, with high-precision 0.0001° step size for omega and 2 θ scans. The storage ring, Helios 2, was running at 700 MeV with typical stored electron beam current of 300 mA. Incident X-ray beam was conditioned to select Cu Kα 1 radiation equivalent (8.048 keV in photon energy) by a Si (111) channel-cut monochromator and toroidal focusing mirror, blocked to be 1.00 mm high in vertical direction and 3.00 mm wide in horizontal direction by a slit system. Such set-up yielded incident X-ray beam with about 0.006° in vertical divergence. The detector slit was adjusted to be 1.00 mm high and 3.00 mm wide. The distance between detector slit and sample centre is about 575 mm. The data for HR-XRD RSM were collected under the framework of ( hkl ) coordinates with precision better than 1/1,000 reciprocal lattice unit. The typical counting time was 1 s for every step of the scans for the mappings. Electrical measurements In-plane transport property of the films was investigated using a PPMS (physical properties measurement system, Quantum Design) at temperatures ranging from 10 to 350 K. Pt electrodes with a 0.4 mm × 0.8 mm were deposited on the LSMO film. Two perpendicular electrode sets (eight electrical leads) were wire-bonded with Ohmic contacts to the two channels (ch1 and ch2) of the PPMS dc resistivity puck. Using this set-up, we measured the temperature dependence of resistivity along the two in-plane directions simultaneously. XAS measurements XAS measurements at Mn L -edge and O K -edge were obtained in total electron yield acquisition mode by recording sample current as a function of photon energy of incident X -rays at the SINS beamline of SSLS in a ultrahigh vacuum chamber with a base pressure of 1 × 10 −10 mbar [24] . Linearly polarized X -ray beam with a degree of polarization better than 90% and energy resolution better than 200 meV was employed for the XAS measurements. The incidence angle ( θ ) of X -rays with respect to the sample surface plane was varied by rotating the polar angle of the sample. All near edge X-ray absorption fine structure (NEXAFS) spectra were normalized by the incident X -ray intensity (I0) monitored by a refocusing mirror to eliminate the fluctuation in the incident X -ray intensity. First-principles calculations Density functional calculations were performed using Perdew-Burke-Ernzerhof parametrization of the generalized gradient approximation (GGA-PBE) to exchange-correlation potential in the density-functional theory as implemented in the VASP code. The projector augmented wave (PAW) pseudopotential was used, where La 5 s 2 5 p 6 5 d 1 6 s 2 , Sr 4 s 2 4 p 6 5 s 2 , Mn 3 p 6 3 d 5 4 s 2 and O 2 s 2 2 p 4 were treated as valence electrons. We used a La 4 Sr 2 Mn 6 O 18 supercell (1 × 3 × 2) to model the La–Sr disordered LSMO alloy ( Fig. 5a ). All calculations were performed with an energy cutoff of 600 eV for the plane wave expansion. Atomic relaxations of the supercell are performed using a 6 × 3 × 3 Monkhorst–Pack grid for k -points sampling and atomic positions are converged until the Hellmann–Feynman forces on each atom are <10 meV Å −1 . The in-plane lattice constant of the supercell is constrained to DSO substrate ( a =3.951 Å and b =3.946 Å), and the out-of-plane lattice parameter is using the corresponding experimental value ( c =3.788 Å). In the density of states calculations, a 12 × 6 × 6 k -points grid is used. The strong electron correlations for Mn 3 d states are considered within the GGA+U approach. We used a value of U eff =6 eV ( U =6 eV and J =0 eV). How to cite this article: Wang, B. et al . Oxygen-driven anisotropic transport in ultra-thin manganite films. Nat. Commun. 4:2778 doi: 10.1038/ncomms3778 (2013).